c-Src and IL-6 inhibit osteoblast differentiation and integrate IGFBP5 signalling Interleukin-6 (IL-6) and c-Src impair osteoblast maturation in vitro and in vivo . Given the similar effects of these factors, they are likely to establish a functional loop to maintain osteoblasts in a less mature status. Here we describe a pathway whereby c-Src stimulates IL-6 expression through the STAT3 factor, which, in response to IL-6 induces insulin-like growth factor 5 (IGFBP5), a c-Src activating factor that amplifies this loop only in immature osteoblasts. In contrast, in mature osteoblasts, IGFBP5 is enhanced by Runx2, but is no longer able to stimulate c-Src activation, as this tyrosine kinase at this stage is downregulated. We find that the IGFBP5 produced by osteoblasts stimulates osteoclastogenesis and bone resorption, acting as an osteoblast–osteoclast coupling factor. Finally, we demonstrate that the integrated actions of c-Src, IL-6 and IGFBP5 also have a role in vivo . We conclude that this pathway is relevant for bone metabolism, both in physiological and in pathological conditions. The family of interleukin (IL)-6-type cytokines comprises IL-6, IL-11, LIF (leukaemia inhibitory factor), OSM (oncostatin M), CNTF (ciliary neurotrophic factor), CT-1 (cardiotrophin-1) and CLC (cardiotrophin-like cytokine) [1] . They activate target genes involved in differentiation, survival, apoptosis and proliferation in several cell types [2] . The members of this cytokine family have pro- as well as anti-inflammatory properties and are major factors in haematopoiesis, and in acute phase and immune responses. The major step in IL-6-type cytokine signalling is the rapid activation of the Janus family tyrosine kinases (JAK proteins) by binding to the signal transducing proteins gp130, LIF receptor and OSM receptor [3] , [4] , [5] . The role played by JAK1 is essential because, in cells lacking JAK1, IL-6 signal transduction is greatly impaired [6] , [7] . The JAK proteins are able to activate the Signal Transducer and Activator of Transcription (STAT) proteins by tyrosine residue phosphorylation [8] , which leads to the formation of active STAT dimers [9] . In response to IL-6 stimulation, STAT proteins rapidly accumulate in the nucleus, where they drive the expression of several genes. IL-6 is a pleiotropic cytokine that has important roles in the inflammatory response [10] . In bone, IL-6 has a well-characterized role in promoting osteoclastogenesis, a physiological process that leads to the generation of the bone-resorbing cells, the osteoclasts [11] . In contrast, IL-6 effects on osteoblasts, the bone cells responsible for bone matrix deposition and mineralization, are quite conflicting and contradictory results have been reported [12] . In our previous work, we characterized the bone phenotype of a prepubertal mouse model, in which IL-6 is expressed at a high level in the bloodstream [13] , demonstrating stunted skeletal growth and osteopenia, with accelerated bone resorption, reduced bone formation and defective ossification. Enhanced bone resorption was due to increased osteoclastogenesis, while reduced osteoblast activity was induced by a mechanism affecting precursor proliferation and mature osteoblast function [13] . A very similar effect on osteoblast function is caused by the activity of c-Src. This is a non-receptor tyrosine kinase, which belongs to a family of cytoplasmic tyrosine kinases (Protein Tyrosine Kinase family, PTKs), capable of communicating with a large number of different receptors [14] , [15] . c-Src activity maintains osteoblasts in a less differentiated status, negatively regulating the expression of differentiation markers [16] . Given the similarity of IL-6 and c-Src effects on osteoblasts, we hypothesized the existence of a functional loop between these two factors, which could provide new insights into the pathogenesis of inflammation-related and other bone diseases. Therefore, in this study we investigated the molecular interactions between IL-6 and c-Src both in in vitro and in multiple animal models, and identified a complex autocrine/paracrine coordination, involving insulin-like growth factor binding protein 5 (IGFBP5), that controls osteoblast differentiation and osteoblast–osteoclast cross-talk. We conclude that this new pathway is essential for bone metabolism, and that its deregulation could contribute to bone disruption in pathological conditions. IL-6 expression is modulated by c-Src signalling The hypothesis of this work arose from a large-scale transcriptome analysis, in which primary mouse calvarial osteoblasts were treated for 24 h with 2 μM of the c-Src inhibitor, PP1. Among several modulated genes, IL-6 expression was >60% reduced versus control (relative expression PP1-treated/vehicle-treated osteoblasts 0.37, n =3, P <0.01, Student's t -test). To validate this result, we replicated the PP1 treatment in a time-course experiment and evaluated IL-6 expression and secretion by reverse transcription–polymerase chain reaction (RT–PCR) and enzyme-linked immunosorbent assay (ELISA), respectively. We confirmed that c-Src inhibition caused a time-dependent decrease of IL-6 mRNA and a consequent reduction of IL-6 accumulation in the conditioned media of our calvarial osteoblast cultures ( Fig. 1a,b ). To further demonstrate our hypothesis, we downregulated the c-Src mRNA by treatment with small interfering RNA (siRNA) and confirmed a reduced IL-6 expression compared with control siRNA ( Fig. 1c ). Similarly, in osteoblasts transfected with a dominant negative (DN), kinase dead, c-Src, reduced c-Src activity decreased IL-6 expression ( Fig. 1d ). In contrast, overexpression of wild-type (WT) c-Src increased IL-6 mRNA ( Fig. 1d ). We therefore concluded that IL-6 expression in osteoblasts is under the control of c-Src. 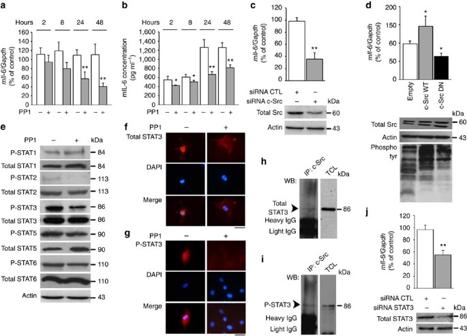Figure 1: c-Src controls IL-6 expression by modulation of STAT3 activation. (a) Mouse calvarial osteoblasts were treated with DMSO or 2 μM PP1 in a time-course experiment. RT–PCR and relative quantification ofIl-6expression, normalized withglyceraldehyde-3-phosphate dehydrogenase(Gapdh) expression (mean±s.d.,n=3, **P<0.01, Student'st-test). (b) ELISA assay of IL-6 protein accumulation in conditioned media in the time-course experiment shown ina(mean±s.d.,n=3, *P<0.05, **P≤0.005, Student'st-test). (c) Mouse calvarial osteoblasts were treated with 100 nM c-Src–siRNA. RT–PCR ofIl-6expression, normalized versusGapdhexpression (mean±s.d.,n=3, **P<0.005, Student'st-test), and western blot (WB) analysis to control total c-Src protein downregulation, normalized versus actin. (d) Mouse calvarial osteoblasts were electroporated with an empty vector, a WT and a dominant negative (DN) variant of c-Src. RT–PCR ofIl-6expression, normalized versusGapdhexpression (mean±s.d.,n=3, *P<0.05, Student'st-test), and WB analysis to control total c-Src protein downregulation and total phospho-tyrosine status, normalized versus actin. (e) STAT proteins, both total and phosphorylated in activating tyrosine residues, were evaluated in DMSO- or PP1-treated osteoblasts, normalized versus actin. (f) Immunofluorescence analysis for total STAT3 in primary mouse osteoblasts treated for 24 h with 2 μM PP1. Results are representative of three independent experiments. Scale bar, 50 μm. (g) Immunofluorescence analysis for phospho-Y705-STAT3 protein in primary mouse osteoblasts treated for 24 h with 2 μM PP1. Results are representative of three independent experiments. Scale bar, 50 μm. (h) Immunoprecipitation (IP) of osteoblast lysates with total c-Src antibody followed by a WB with a total STAT3 antibody. Results are representative of three independent experiments. TCL, total cell lysate. (i) Stripping of the membrane shown inhand staining with a P-Y705-STAT3 antibody. (j) Mouse calvarial osteoblasts were treated with 100 nM STAT3–siRNA. RT–PCR ofIl-6expression, normalized versusGapdh(mean±s.d.,n=3, **P<0.005, Student'st-test), and WB analysis to control total c-Src protein downregulation, normalized versus actin. CTL, control siRNA; DAPI, 4,6-diamidino-2-phenylindole; IgG, immunoglobulin-G. Figure 1: c-Src controls IL-6 expression by modulation of STAT3 activation. ( a ) Mouse calvarial osteoblasts were treated with DMSO or 2 μM PP1 in a time-course experiment. RT–PCR and relative quantification of Il-6 expression, normalized with glyceraldehyde-3-phosphate dehydrogenase ( Gapdh ) expression (mean±s.d., n =3, ** P <0.01, Student's t -test). ( b ) ELISA assay of IL-6 protein accumulation in conditioned media in the time-course experiment shown in a (mean±s.d., n =3, * P <0.05, ** P ≤0.005, Student's t -test). ( c ) Mouse calvarial osteoblasts were treated with 100 nM c-Src–siRNA. RT–PCR of Il-6 expression, normalized versus Gapdh expression (mean±s.d., n =3, ** P <0.005, Student's t -test), and western blot (WB) analysis to control total c-Src protein downregulation, normalized versus actin. ( d ) Mouse calvarial osteoblasts were electroporated with an empty vector, a WT and a dominant negative (DN) variant of c-Src. RT–PCR of Il-6 expression, normalized versus Gapdh expression (mean±s.d., n =3, * P <0.05, Student's t -test), and WB analysis to control total c-Src protein downregulation and total phospho-tyrosine status, normalized versus actin. ( e ) STAT proteins, both total and phosphorylated in activating tyrosine residues, were evaluated in DMSO- or PP1-treated osteoblasts, normalized versus actin. ( f ) Immunofluorescence analysis for total STAT3 in primary mouse osteoblasts treated for 24 h with 2 μM PP1. Results are representative of three independent experiments. Scale bar, 50 μm. ( g ) Immunofluorescence analysis for phospho-Y705-STAT3 protein in primary mouse osteoblasts treated for 24 h with 2 μM PP1. Results are representative of three independent experiments. Scale bar, 50 μm. ( h ) Immunoprecipitation (IP) of osteoblast lysates with total c-Src antibody followed by a WB with a total STAT3 antibody. Results are representative of three independent experiments. TCL, total cell lysate. ( i ) Stripping of the membrane shown in h and staining with a P-Y705-STAT3 antibody. ( j ) Mouse calvarial osteoblasts were treated with 100 nM STAT3–siRNA. RT–PCR of Il-6 expression, normalized versus Gapdh (mean±s.d., n =3, ** P <0.005, Student's t -test), and WB analysis to control total c-Src protein downregulation, normalized versus actin. CTL, control siRNA; DAPI, 4,6-diamidino-2-phenylindole; IgG, immunoglobulin-G. Full size image c-Src regulates IL-6 expression through STAT3 Because c-Src is not a transcription factor, we wondered what molecular mechanism could be involved in the regulation of IL-6 expression. Therefore, we analysed data from the gene profile of PP1-treated osteoblasts, using the web-based platform Gene Ontology Tree Machine and noted that the JAK/STAT signalling pathway was significantly downregulated in PP1-treated osteoblasts versus control. We hence verified if c-Src phosphorylates members of the STAT transcription factor family analysing their activating phosphorylation status in osteoblasts treated with PP1. Small or no differences were observed in the activation of STAT proteins, except for phospho-Y-705-STAT3, which was strongly decreased by the treatment with PP1 ( Fig. 1e ). To confirm the involvement of STAT3, we performed immunofluorescence analysis and demonstrated that in basal condition most STAT3 protein was concentrated in and around the nucleus, indicating its active status, while in c-Src inhibitor-treated osteoblasts, STAT3 was mainly localized in the cytoplasm ( Fig. 1f ), presumably in an inactive form. Consistent with this, using an antibody recognizing the phospho-Y-705-STAT3, we confirmed that c-Src inhibition caused a reduction in STAT3-activating phosphorylation ( Fig. 1g ). To assess whether c-Src and STAT3 physically interacted, we performed immunoprecipitation assay and demonstrated that indeed c-Src coimmunoprecipitated with STAT3 ( Fig. 1h ) in a complex in which STAT3 was in the active phosphorylated status ( Fig. 1i ). Finally, to confirm the functional link between STAT3 and IL-6, we downregulated STAT3 mRNA by treatment with siRNA and observed the expected reduction of IL-6 mRNA expression ( Fig. 1j ). Taken together, these results indicate that c-Src and STAT3 could converge in the regulation of IL-6 transcription. STAT3 and c-Src have similar roles on osteoblast function We next asked whether STAT3 has a role in c-Src activation, through which it could affect osteoblast differentiation. To this end, we silenced STAT3 mRNA by treatment with siRNA and saw a concentration-dependent decrease of c-Src activating phosphorylation ( Fig. 2a ), indicating that these two pathways are closely interrelated and modulate each other. To verify whether this interaction affected osteoblast differentiation, in STAT3 mRNA downregulated osteoblasts, we investigated the transcriptional expression of osteoblast-specific markers and observed an increase in Runx2 , Collagen 1A2 and Osteocalcin ( Fig. 2b ), demonstrating the inverse correlation between this IL-6 upstream signal and osteoblast differentiation. Notably, this result was very similar to the well-known effect of c-Src downregulation on osteoblast differentiation [16] . In fact, we found comparable upregulation of these osteoblast-specific genes in osteoblasts treated with c-Src–siRNA ( Fig. 2c ). To assess whether IL-6, whose receptor is up-stream of STAT3, inhibited osteoblast differentiation, we treated primary mouse osteoblasts with rhIL-6 and observed a reduction in Runx2 , Collagen 1A2 and Osteocalcin expression that was reversed by treatment with an anti-IL-6 antibody ( Fig. 2d ). This latter treatment increased Runx2 , Collagen 1A2 and Osteocalcin above the control levels. To verify whether this event reflected the presence in our cultures of endogenous mouse IL-6 autocrinely produced by the osteoblasts, we performed an ELISA assay in the supernatants and noted a marked reduction of IL-6 protein in the presence of the antibody ( Fig. 2e ). 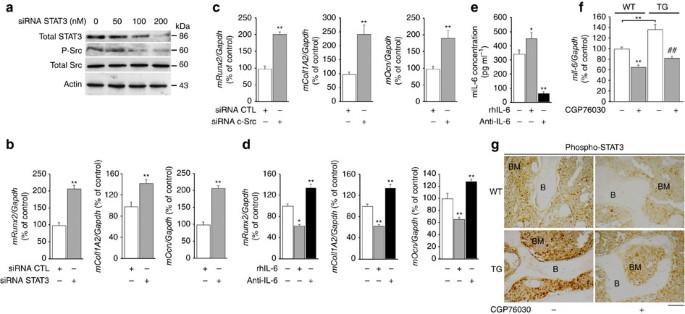Figure 2: Feedback regulation between IL-6 and c-Src signalsin vitroandin vivo. (a) Mouse calvarial osteoblasts were treated with control siRNA (0) or increasing concentrations of STAT3–siRNA. Western Blot analysis of total STAT3 protein, c-Src activating phosphorylation and total Src protein, normalized versus actin. (b) RT–PCR of the indicated osteoblast differentiation markers in osteoblasts treated with control siRNA or STAT3–siRNA, normalized versusglyceraldehyde-3-phosphate dehydrogenase(Gapdh; mean±s.d.,n=3, **P<0.005, Student'st-test). (c) Osteoblast differentiation marker expression assessed by RT–PCR in osteoblasts treated with control siRNA or c-Src–siRNA, normalized versusGapdh(mean±s.d.,n=3, **P<0.005, Student'st-test). (d) Mouse calvarial osteoblasts were cultured for 24 h in the presence of vehicle, 5 ng ml−1of rhIL-6 or 1 μg ml−1of anti-IL-6 antibody. Osteoblast differentiation marker expression was assessed by RT–PCR, normalized versusGapdh(mean±s.d.,n=3, **P<0.005, Student'st-test). (e) ELISA assay of endogenous (mouse) IL-6 protein accumulation in conditioned media of rhIL-6- or anti-IL-6-treated osteoblasts (mean±s.d.,n=3, *P<0.05; **P<0.001, Student'st-test). (f) Eight-week-old WT and NSE/hIL-6 (TG) mice were treated for 1 month with 100 mg kg−1per day of the c-Src inhibitor CGP76030 by oral gavage. Relative quantification of IL-6 mRNA expression, normalized withGapdh, in RNA extracted from tibias (mean±s.d.,n=3, **P<0.005 versus vehicle-treated WT mice.##P<0.005 versus vehicle-treated TG mice, Student'st-test). (g) Immunohistochemistry in paraffin-embedded 5-μm-thick tibias sections of WT and TG mice treated with CGP76030 inhibitor. Staining for phospho-Y705-STAT3. B, bone; BM, bone marrow. Scale bar, 50 μm. Figure 2: Feedback regulation between IL-6 and c-Src signals in vitro and in vivo . ( a ) Mouse calvarial osteoblasts were treated with control siRNA (0) or increasing concentrations of STAT3–siRNA. Western Blot analysis of total STAT3 protein, c-Src activating phosphorylation and total Src protein, normalized versus actin. ( b ) RT–PCR of the indicated osteoblast differentiation markers in osteoblasts treated with control siRNA or STAT3–siRNA, normalized versus glyceraldehyde-3-phosphate dehydrogenase ( Gapdh ; mean±s.d., n =3, ** P <0.005, Student's t -test). ( c ) Osteoblast differentiation marker expression assessed by RT–PCR in osteoblasts treated with control siRNA or c-Src–siRNA, normalized versus Gapdh (mean±s.d., n =3, ** P <0.005, Student's t -test). ( d ) Mouse calvarial osteoblasts were cultured for 24 h in the presence of vehicle, 5 ng ml −1 of rhIL-6 or 1 μg ml −1 of anti-IL-6 antibody. Osteoblast differentiation marker expression was assessed by RT–PCR, normalized versus Gapdh (mean±s.d., n =3, ** P <0.005, Student's t -test). ( e ) ELISA assay of endogenous (mouse) IL-6 protein accumulation in conditioned media of rhIL-6- or anti-IL-6-treated osteoblasts (mean±s.d., n =3, * P <0.05; ** P <0.001, Student's t -test). ( f ) Eight-week-old WT and NSE/hIL-6 (TG) mice were treated for 1 month with 100 mg kg −1 per day of the c-Src inhibitor CGP76030 by oral gavage. Relative quantification of IL-6 mRNA expression, normalized with Gapdh , in RNA extracted from tibias (mean±s.d., n =3, ** P <0.005 versus vehicle-treated WT mice. ## P <0.005 versus vehicle-treated TG mice, Student's t -test). ( g ) Immunohistochemistry in paraffin-embedded 5-μm-thick tibias sections of WT and TG mice treated with CGP76030 inhibitor. Staining for phospho-Y705-STAT3. B, bone; BM, bone marrow. Scale bar, 50 μm. Full size image Interplay between c-Src and IL-6 in vivo To investigate the significance of the interplay between c-Src and IL-6 on bone in vivo , we evaluated the IL-6 mRNA expression in WT and IL-6 transgenic (TG) mice, overexpressing human IL-6 in the circulation and treated with the pharmacological c-Src inhibitor, substituted 5,7-diphenyl-pyrrolo[2,3- d ]-pyrimidine, CGP76030 (ref. 17 ). As in the TG mice the human IL-6 transgene is constitutively overexpressed and, therefore, not regulated, we analysed the expression of the endogenous (mouse) IL-6. c-Src inhibition caused a reduction of mouse IL-6 mRNA expression in tibias of WT mice ( Fig. 2f ). Notably, in the IL-6 TG mice, overexpressed human IL-6 induced endogenous mouse IL-6 expression in bone, and this induction was also prevented by c-Src inhibition ( Fig. 2f ). To assess the role of STAT3 in this context, we performed immunohistochemical analysis on femurs of WT and IL-6 TG mice and demonstrated reduced levels of activated STAT3 after treatment with the c-Src inhibitor, more evident in IL-6 TG mice in which, possibly due to the IL-6 overexpression, STAT3 basal activation was higher than in WT mice ( Fig. 2g ). These results indicate that c-Src regulates IL-6 expression in vivo through STAT3. Role of the interplay between c-Src and IL-6 in bone metabolism To examine the role played by the interplay between c-Src and IL-6 on bone metabolism in vivo , we investigated the bone phenotype of WT and IL-6 TG mice treated with the c-Src inhibitor CGP76030. Serum levels or mRNA expression in bone of the osteoblast markers Osteocalcin ( Fig. 3a,b ), Runx2 ( Fig. 3c ) and Collagen 1A2 ( Fig. 3d ) were upregulated in both WT and IL-6 TG mice by c-Src inhibition, further indicating an increase in osteoblast activity. In contrast, the serum levels of the osteoclast marker, TRAcP-5b ( Fig. 3e ), and of the bone resorption marker, C-terminal fragment of Collagen I ( Fig. 3f ), were downregulated in both WT and IL-6 TG mice treated with CGP76030. Histomorphometric analysis performed on femurs showed that the treatment with CGP76030 slightly increased the bone structural parameters of WT mice and had a robust effect in TG mice, in which it strongly increased the bone volume and the trabecular parameters of the secondary spongiosa ( Fig. 3g ), significantly improving their bone phenotype. Analysis of cellular parameters demonstrated the anabolic and the antiresorptive effects of the c-Src inhibitor, which affected osteoblast activity ( Fig. 3h,i ), mineral deposition ( Fig. 3j ) and osteoclast parameters ( Fig. 3h and Supplementary Fig. S1 ), especially in IL-6 TG mice. These data indicate that c-Src exerts a role on the IL-6-induced osteopenic phenotype in vivo . 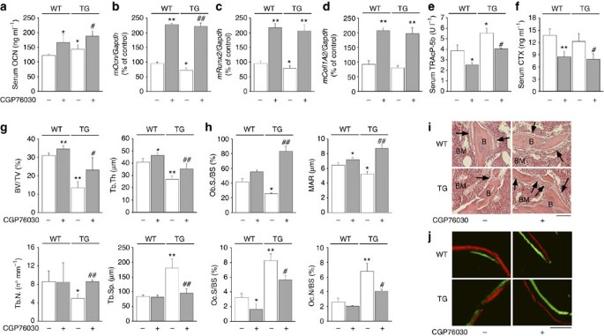Figure 3: c-Src/IL-6 interplay in bone metabolism. Eight-week-old WT and NSE/hIL-6 TG mice were treated for 1 month with vehicle (tartaric acid) or 100 mg kg−1per day of the c-Src inhibitor CGP76030. (a) ELISA assay for osteocalcin (OCN) detection in sera. (b) RT–PCR and relative quantification ofOcnexpression in tibias, normalized toGapdh. (c) RT–PCR and relative quantification ofRunx2expression in tibias, normalized toGapdh. (d) RT–PCR and relative quantification ofCol1A2expression in tibias, normalized toGapdh. (e) ELISA assay for TRAcP-5b detection in sera. (f) ELISA assay for C-terminal fragment of Collagen I (CTX) detection in sera. Histomorphometric analysis showing (g) the structural parameters bone volume/total volume (BV/TV), trabecular thickness (Tb.Th.), trabecular number (Tb.N.) and trabecular separation (Tb.Sp.), and (h) the cellular and the dynamic parameters osteoblast surface (Ob.S/BS), mineral apposition rate (MAR), osteoclast surface (Oc.S/BS) and osteoclast number (Oc.N/BS). Mean±s.d.;n=3–5 animals per group. *P<0.05 and **P<0.005 versus vehicle-treated WT mice.#P<0.05 and##P<0.005 versus vehicle-treated TG mice, Student'st-test. (i) Haematoxylin/eosin staining of paraffin-embedded 5-μm-thick femur sections of vehicle-and CGP76030-treated mice. Arrows, osteoblasts on trabecular bone. B, bone; BM, bone marrow. Scale bar, 50 μm. (j) Doublein vivoalizarin red S (red fluorescence) and calcein (green fluorescence) labelling of methacrylate-embedded femur sections from vehicle- and CGP76030-treated mice. Scale bar, 50 μm.Gapdh,glyceraldehyde-3-phosphate dehydrogenase. Figure 3: c-Src/IL-6 interplay in bone metabolism. Eight-week-old WT and NSE/hIL-6 TG mice were treated for 1 month with vehicle (tartaric acid) or 100 mg kg −1 per day of the c-Src inhibitor CGP76030. ( a ) ELISA assay for osteocalcin (OCN) detection in sera. ( b ) RT–PCR and relative quantification of Ocn expression in tibias, normalized to Gapdh . ( c ) RT–PCR and relative quantification of Runx2 expression in tibias, normalized to Gapdh . ( d ) RT–PCR and relative quantification of Col1A2 expression in tibias, normalized to Gapdh . ( e ) ELISA assay for TRAcP-5b detection in sera. ( f ) ELISA assay for C-terminal fragment of Collagen I (CTX) detection in sera. Histomorphometric analysis showing ( g ) the structural parameters bone volume/total volume (BV/TV), trabecular thickness (Tb.Th. ), trabecular number (Tb.N.) and trabecular separation (Tb.Sp. ), and ( h ) the cellular and the dynamic parameters osteoblast surface (Ob.S/BS), mineral apposition rate (MAR), osteoclast surface (Oc.S/BS) and osteoclast number (Oc.N/BS). Mean±s.d. ; n =3–5 animals per group. * P <0.05 and ** P <0.005 versus vehicle-treated WT mice. # P <0.05 and ## P <0.005 versus vehicle-treated TG mice, Student's t -test. ( i ) Haematoxylin/eosin staining of paraffin-embedded 5-μm-thick femur sections of vehicle-and CGP76030-treated mice. Arrows, osteoblasts on trabecular bone. B, bone; BM, bone marrow. Scale bar, 50 μm. ( j ) Double in vivo alizarin red S (red fluorescence) and calcein (green fluorescence) labelling of methacrylate-embedded femur sections from vehicle- and CGP76030-treated mice. Scale bar, 50 μm. Gapdh , glyceraldehyde-3-phosphate dehydrogenase . Full size image Role of the interplay between c-Src and IL-6 in inflammation IL-6 is an important cytokine with a prominent role in many inflammatory diseases. To investigate the significance of the interplay between c-Src and IL-6 on the inflammatory response, WT mice were pretreated for 24 h with CGP76030 and the subsequent day they received the inflammation-inducing agent, lipopolysaccharide (LPS). We evaluated IL-6 mRNA in the whole tibias 6 h after LPS administration and, as expected, we found an increased expression compared with vehicle-treated animals. In contrast, in mice treated with the c-Src inhibitor this induction was significantly hampered ( Fig. 4a ). To induce a specific IL-6-mediated inflammation, we also pretreated the mice for 24 h with CGP76030, followed by turpentine for 6 h. Once again, induction of IL-6 mRNA by turpentine was inhibited in tibias of CGP76030-treated mice ( Fig. 4a ), confirming that, in vivo , c-Src not only controls IL-6 expression in bone but also in inflammatory conditions. To confirm that the inflammatory response was induced in the mice, we tested two other mediators of inflammation, IL-1β and tumour-necrosis factor-α, which were upregulated by our proinflammatory stimuli ( Fig. 4a ). Interestingly, while tumour-necrosis factor-α was insensitive to the treatment with CGP76030, IL-1β, which is known to be induced by IL-6 itself [13] , was subjected to similar downregulation by CGP76030 as IL-6. 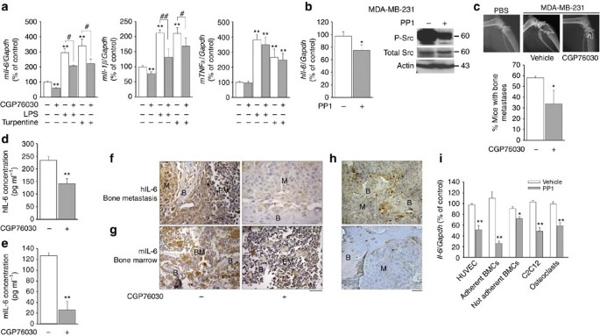Figure 4: IL-6/c-Src interplay inin vivopathological conditions. (a) Eight-week-old mice were treated for 24 h with 100 mg kg−1per day c-Src inhibitor and then for 6 h with vehicle (PBS), LPS (2.5 μg per mouse) or turpentine (100 μl per mouse). RT–PCR and relative quantification ofIl-6expression (mean±s.d.;n=3; **P<0.001 versus vehicle-treated mice.#P<0.001 versus anti-inflammatory agent-treated mice, Student'st-test),Il-1βexpression (mean±s.d.;n=3; *P<0.05 and **P<0.01 versus vehicle-treated mice.#P<0.05 and##P<0.005 versus anti-inflammatory agent-treated mice, Student'st-test) andtumour-necrosis factor-αexpression (mean±s.d.;n=3; *P<0.05 and **P<0.01 versus vehicle-treated mice.#P<0.05 and##P<0.005 versus anti-inflammatory agent-treated mice, Student'st-test) in tibias, normalized withGapdh. (b) Human breast cancer MDA-MB-231 cells were treated with 2 μM PP1 for 24 h. RT–PCR of humanIl-6expression, normalized versusGapdhexpression (mean±s.d.,n=3, *P<0.05, Student'st-test) and western blot analysis to control total c-Src protein downregulation and activating phosphorylation, normalized versus actin. (c) Four-week-old female BALB/c-nu/numice intracardiacally injected with PBS or with a suspension (100,000 cells per 100 μl of PBS) of MDA-MB-231 cells. X-ray images and incidence of bone metastasis in mice treated with vehicle or with the c-Src inhibitor CGP76030 (100 mg kg−1per day) for 38 days; in X-ray imagine bone metastases are delineated by a white line.N=8 animals per group. ELISA assay for (d) human and (e) mouse IL-6 in the sera of mice carrying MDA-MB-231 cell-induced bone metastases treated with vehicle or with the c-Src inhibitor CGP76030 (100 mg kg−1per day) for 38 days after intracardiac tumour cell injection. Mean±s.d.;n=3; **P<0.005, Student'st-test. Immunohistochemical staining for (f) human IL-6 (scale bar, 50 μm) and (g) mouse IL-6 (scale bar, 50 μm) in paraffin-embedded 5-μm-thick tibia sections of MDA-MB-231 cell-injected mice treated with the CGP76030 inhibitor. (h) Control of species-specificity of anti-mouse and anti-human IL-6 antibodies in the metastatic tissue. Scale bar, 50 μm. B, bone; BM, bone marrow; M, metastasis. (i) RT–PCR forIl-6expression in the indicated cells treated with 2 μM PP1, normalized versusGapdh(mean±s.d.,n=3. *P<0.05 and **P<0.005, Student'st-test).Gapdh,glyceraldehyde-3-phosphate dehydrogenase; HUVEC, human umbilical vein endothelial cell. Figure 4: IL-6/c-Src interplay in in vivo pathological conditions. ( a ) Eight-week-old mice were treated for 24 h with 100 mg kg −1 per day c-Src inhibitor and then for 6 h with vehicle (PBS), LPS (2.5 μg per mouse) or turpentine (100 μl per mouse). RT–PCR and relative quantification of Il-6 expression (mean±s.d. ; n =3; ** P <0.001 versus vehicle-treated mice. # P <0.001 versus anti-inflammatory agent-treated mice, Student's t -test), Il-1β expression (mean±s.d. ; n =3; * P <0.05 and ** P <0.01 versus vehicle-treated mice. # P <0.05 and ## P <0.005 versus anti-inflammatory agent-treated mice, Student's t -test) and tumour-necrosis factor-α expression (mean±s.d. ; n =3; * P <0.05 and ** P <0.01 versus vehicle-treated mice. # P <0.05 and ## P <0.005 versus anti-inflammatory agent-treated mice, Student's t -test) in tibias, normalized with Gapdh . ( b ) Human breast cancer MDA-MB-231 cells were treated with 2 μM PP1 for 24 h. RT–PCR of human Il-6 expression, normalized versus Gapdh expression (mean±s.d., n =3, * P <0.05, Student's t -test) and western blot analysis to control total c-Src protein downregulation and activating phosphorylation, normalized versus actin. ( c ) Four-week-old female BALB/c- nu/nu mice intracardiacally injected with PBS or with a suspension (100,000 cells per 100 μl of PBS) of MDA-MB-231 cells. X-ray images and incidence of bone metastasis in mice treated with vehicle or with the c-Src inhibitor CGP76030 (100 mg kg −1 per day) for 38 days; in X-ray imagine bone metastases are delineated by a white line. N =8 animals per group. ELISA assay for ( d ) human and ( e ) mouse IL-6 in the sera of mice carrying MDA-MB-231 cell-induced bone metastases treated with vehicle or with the c-Src inhibitor CGP76030 (100 mg kg −1 per day) for 38 days after intracardiac tumour cell injection. Mean±s.d. ; n =3; ** P <0.005, Student's t -test. Immunohistochemical staining for ( f ) human IL-6 (scale bar, 50 μm) and ( g ) mouse IL-6 (scale bar, 50 μm) in paraffin-embedded 5-μm-thick tibia sections of MDA-MB-231 cell-injected mice treated with the CGP76030 inhibitor. ( h ) Control of species-specificity of anti-mouse and anti-human IL-6 antibodies in the metastatic tissue. Scale bar, 50 μm. B, bone; BM, bone marrow; M, metastasis. ( i ) RT–PCR for Il-6 expression in the indicated cells treated with 2 μM PP1, normalized versus Gapdh (mean±s.d., n =3. * P <0.05 and ** P <0.005, Student's t -test). Gapdh , glyceraldehyde-3-phosphate dehydrogenase ; HUVEC, human umbilical vein endothelial cell. Full size image Role of the interplay between c-Src and IL-6 in bone metastases Breast cancer bone metastases are inhibited by c-Src inactivation due to its antiresorptive and antiproliferative effects [17] . To assess whether this condition influenced IL-6 metabolism, we evaluated IL-6 in mice carrying bone metastases induced by the human breast cancer MDA-MB-231 cells. In vitro , these cells showed reduced IL-6 mRNA expression when treated with the c-Src inhibitor PP1 ( Fig. 4b ). BALB/c- nu/nu mice were subjected to intracardiac injection of MDA-MB-231 cells and treated with CGP76030, which, as expected, significantly reduced the incidence of bone metastases compared with untreated mice [17] ( Fig. 4c ). This treatment also caused a reduction of both the human (derived by MDA-MB-231 cells) and the mouse IL-6 by c-Src inhibition detected both in sera ( Fig. 4d,e ) and in the bone metastasis tissue ( Fig. 4f–h ). Role of the interplay between c-Src and IL-6 in other cell types Having noted in Figure 4f,g that IL-6 expression was impaired by c-Src inhibition in various cell types, we further investigated whether the interplay between IL-6 and c-Src was typical of cells from different tissues. Indeed, we confirmed the c-Src-mediated regulation of IL-6 expression in a panel of primary cells and established cell lines ( Fig. 4i ), supporting the idea that the interplay described in this work is a general mechanism with a systemic relevance. IL-6 signal activates c-Src through the IGFBP5 pathway We next asked whether IL-6 could impact c-Src, thus creating a loop of regulation. To this purpose, we treated primary mouse osteoblasts with hrIL-6 and observed a time-dependent increase in the phosphorylation of c-Src Y-416, which only became robust after long-term treatments (8 days; Fig. 5a ), suggesting the involvement of intermediate factors. Among several candidate proteins, the insulin-like growth factor-1 (IGF-1) could be instrumental in linking the IL-6 and c-Src pathways, given that the IGF-1 receptor is able to induce c-Src activation [18] . However, in primary mouse osteoblasts treated with rhIL-6 for 1 week we found no effect on IGF-1 mRNA content ( Fig. 5b ). Because the effects of IGF-1 are under the control of various IGFBPs, we tested a panel of IGFBPs and observed upregulation of IGFBP5 mRNA compared with control cultures ( Fig. 5c ). In addition, IGFBP5 mRNA expression was inhibited when the IL-6-sensitive transcription factor STAT3 was downregulated by treatment with siRNA ( Fig. 5d ). To assess whether IGFBP5 signalled through c-Src, we treated primary mouse osteoblasts for 30 min with increasing concentrations of soluble IGFBP5 and observed a concentration-dependent increase of c-Src Y-416 activating phosphorylation ( Fig. 5e ). To our surprise, this effect was independent of the IGF-1 receptor signal because the treatment with IGFBP5 did not increase its activating phosphorylation ( Fig. 5e ). To address the link between c-Src and IGFBP5 expression, we downregulated the IGFBP5 by siRNA and noted a consistent reduction of the c-Src Y-416 activating phosphorylation compared with control siRNA ( Fig. 5f ). Taken together, these observations indicated an IGF1-independent functional role for IGFBP5 in the interplay between IL-6 and c-Src in osteoblasts. 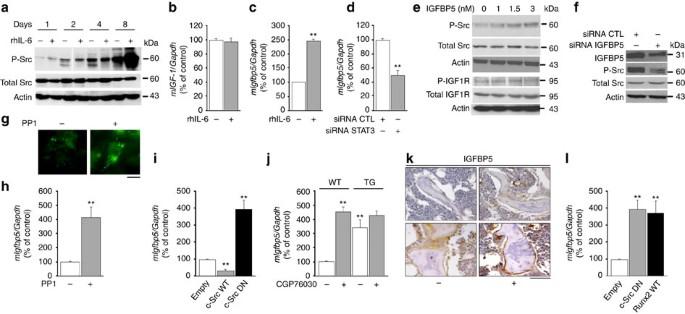Figure 5: IGFBP5 involvement in the IL-6-dependent c-Src activation. (a) Mouse calvarial osteoblasts were treated with vehicle (acetic acid) or with 5 ng ml−1rhIL-6 in a time-course experiment. Western blot analysis of c-Src activating phosphorylation and total c-Src, normalized versus actin. (b) RT–PCR for IGF-1 expression in osteoblasts treated with 5 ng ml−1rhIL-6, normalized versusGapdh(mean±s.d.,n=3). (c) RT–PCR forIgfbp5expression in osteoblasts treated with 5 ng ml−1rhIL-6, normalized versusGapdh(mean±s.d.,n=3, **P<0.005, Student'st-test). (d) RT–PCR forIgfbp5expression in primary osteoblasts treated with 100 nM of control siRNA (CTL) or siRNA for STAT3, normalized toGapdh(mean±s.d.,n=3, **P<0.005, Student'st-test). (e) Mouse calvarial osteoblasts were treated with the indicated concentrations of soluble IGFBP5 for 30 min. Western blot analysis of c-Src and IGF-1 receptor (IGF1R) activating phosphorylation, normalized versus the respective total proteins and actin. (f) Mouse calvarial osteoblasts were treated with 100 nM of control siRNA (CTL) or siRNA–IGFBP5. Western blot analysis of IGFBP5 and of c-Src activating phosphorylation, normalized versus the respective total proteins and actin. (g) Immunostaining analysis for IGFBP5 in primary mouse osteoblasts treated for 24 h with vehicle (DMSO) or 2 μM PP1. Scale bar, 50 μm. (h) RT–PCR forIgfbp5, normalized versusGapdhexpression (mean±s.d.,n=3, **P<0.005, Student'st-test). (i) RT–PCR forIgfbp5in primary mouse osteoblasts transfected with an empty vector (as a control) and WT and DN c-Src variants, normalized versusGapdhexpression (mean±s.d.,n=3, **P<0.005, Student'st-test). (j) Relative quantification ofIgfbp5mRNA expression, normalized withGapdh, in RNA extracted from tibias of eight week-old WT and NSE/hIL-6 (TG) mice treated for 1 month with 100 mg kg−1per day of the c-Src inhibitor CGP76030 (mean±s.d.,n=3, **P<0.005, Student'st-test). (k) Immunohistochemistry for IGFBP5 in paraffin-embedded 5-μm-thick tibia sections of WT and TG mice treated with vehicle or with the CGP76030 inhibitor. B, bone; BM, bone marrow. Scale bar, 50 μm. (l) RT–PCR forIgfbp5in primary mouse osteoblasts transfected with an empty vector (as a control), c-Src DN and Runx2 WT vectors, normalized toGapdhexpression (mean±s.d.,n=3, **P<0.005, Student'st-test).Gapdh,glyceraldehyde-3-phosphate dehydrogenase. Figure 5: IGFBP5 involvement in the IL-6-dependent c-Src activation. ( a ) Mouse calvarial osteoblasts were treated with vehicle (acetic acid) or with 5 ng ml −1 rhIL-6 in a time-course experiment. Western blot analysis of c-Src activating phosphorylation and total c-Src, normalized versus actin. ( b ) RT–PCR for IGF-1 expression in osteoblasts treated with 5 ng ml −1 rhIL-6, normalized versus Gapdh (mean±s.d., n =3). ( c ) RT–PCR for Igfbp5 expression in osteoblasts treated with 5 ng ml −1 rhIL-6, normalized versus Gapdh (mean±s.d., n =3, ** P <0.005, Student's t -test). ( d ) RT–PCR for Igfbp5 expression in primary osteoblasts treated with 100 nM of control siRNA (CTL) or siRNA for STAT3, normalized to Gapdh (mean±s.d., n =3, ** P <0.005, Student's t -test). ( e ) Mouse calvarial osteoblasts were treated with the indicated concentrations of soluble IGFBP5 for 30 min. Western blot analysis of c-Src and IGF-1 receptor (IGF1R) activating phosphorylation, normalized versus the respective total proteins and actin. ( f ) Mouse calvarial osteoblasts were treated with 100 nM of control siRNA (CTL) or siRNA–IGFBP5. Western blot analysis of IGFBP5 and of c-Src activating phosphorylation, normalized versus the respective total proteins and actin. ( g ) Immunostaining analysis for IGFBP5 in primary mouse osteoblasts treated for 24 h with vehicle (DMSO) or 2 μM PP1. Scale bar, 50 μm. ( h ) RT–PCR for Igfbp5 , normalized versus Gapdh expression (mean±s.d., n =3, ** P <0.005, Student's t -test). ( i ) RT–PCR for Igfbp5 in primary mouse osteoblasts transfected with an empty vector (as a control) and WT and DN c-Src variants, normalized versus Gapdh expression (mean±s.d., n =3, ** P <0.005, Student's t -test). ( j ) Relative quantification of Igfbp5 mRNA expression, normalized with Gapdh , in RNA extracted from tibias of eight week-old WT and NSE/hIL-6 (TG) mice treated for 1 month with 100 mg kg −1 per day of the c-Src inhibitor CGP76030 (mean±s.d., n =3, ** P <0.005, Student's t -test). ( k ) Immunohistochemistry for IGFBP5 in paraffin-embedded 5-μm-thick tibia sections of WT and TG mice treated with vehicle or with the CGP76030 inhibitor. B, bone; BM, bone marrow. Scale bar, 50 μm. ( l ) RT–PCR for Igfbp5 in primary mouse osteoblasts transfected with an empty vector (as a control), c-Src DN and Runx2 WT vectors, normalized to Gapdh expression (mean±s.d., n =3, ** P <0.005, Student's t -test). Gapdh , glyceraldehyde-3-phosphate dehydrogenase . Full size image c-Src has an unexpected inhibitory effect on Igfbp5 expression As IL-6 activates c-Src ( Fig. 5a ) and increases IGFBP5 mRNA ( Fig. 5c ), we expected an impairment of IGFBP5 expression in PP1-treated osteoblasts. To our surprise, analysing our global gene profiling, we observed that c-Src inhibition induced a 4.95-fold increase of Igfbp5 gene expression over vehicle-treated osteoblasts. This unexpected result was also confirmed by immunofluorescence analysis ( Fig. 5g ) and RT–PCR ( Fig. 5h ). To ensure that this was not a technical problem, we also overexpressed the WT or a DN form of c-Src in osteoblasts and confirmed that, while WT c-Src reduced IGFBP5 expression, the DN form increased the IGFBP5 mRNA ( Fig. 5i ). The c-Src- and IL-6-mediated regulation of Igfbp5 expression was also confirmed in vivo in WT and IL-6 TG mice. Indeed, in the tibia of WT mice treated with the c-Src inhibitor CGP76030, we revealed a significant induction of the Igfbp5 mRNA expression ( Fig. 5j ). Interestingly, the IL-6 TG mice had a high basal level of IGFBP5 mRNA compared with WT mice ( Fig. 5j ), which was modestly increased by the c-Src inhibition. These findings were also confirmed at the protein level by immunohistochemistry ( Fig. 5k ). To identify a putative molecular mechanism that could explain this unexpected observation, we analysed the promoter sequence of the IGFBP5 gene with the GENOMATIX software that recognizes responsive elements for various transcription factors and identified a responsive element for Runx2, a transcription factor indispensable for osteoblast differentiation that we had found significantly upregulated in c-Src-inhibited osteoblasts (see Fig. 2c ). To determine the role of Runx2, we overexpressed the gene in osteoblasts and assessed the IGFBP5 mRNA expression by RT–PCR comparing the effect with the c-Src inhibition obtained by transfection of the DN c-Src vector. We found that, similar to the DN c-Src, Runx2 overexpression induced IGFBP5 mRNA upregulation ( Fig. 5l ). Therefore, Runx2 could represent the link between c-Src and IGFBP5 operating as a loop alternative to the c-Src/IL-6 pathway to balance the excess of IL-6 activity in osteoblasts. To further examine this putative alternative loop, we wondered whether the effects of IGFBP5 on c-Src could be related to the status of osteoblast maturation. To this purpose, IGFBP5 was administered to osteoblasts at subconfluence, a condition in which cells are immature and proliferating, and at overconfluence, a condition in which osteoblast maturation is complete and cells produce mineralizing osteoid. We observed that c-Src was highly expressed and its activating Y-416 was phosphorylated by the IGFBP5 when the cells were at subconfluence ( Fig. 6a ), while in overconfluent osteoblasts c-Src was barely expressed and, therefore, hardly sensitive to IGFBP5-induced phosphorylation ( Fig. 6b ). 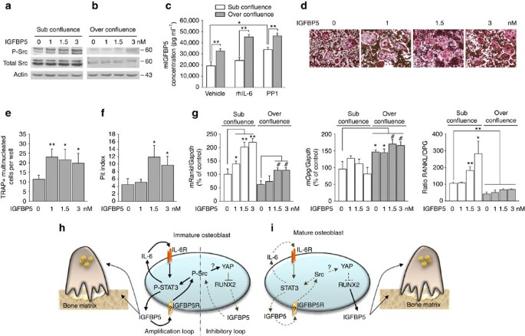Figure 6: IGFBP5 effects on osteoblasts and osteoclasts. (a) Mouse calvarial osteoblasts were cultured at subconfluence and treated with the indicated concentrations of soluble IGFBP5 for 30 min. Western blot analysis of c-Src activating phosphorylation and total c-Src protein, normalized versus actin. (b) Mouse calvarial osteoblasts were cultured at overconfluence and treated with the indicated concentrations of soluble IGFBP5 for 30 min. Western blot analysis of c-Src activating phosphorylation and total c-Src protein, normalized versus actin. (c) ELISA assay for mIGFBP5 detection in the conditioned media from sub- and overconfluent osteoblasts treated with 5 ng ml−1rhIL-6 or with 2 μM PP1 (mean±s.d.,n=3. *P<0.05 and **P<0.005, Student'st-test). (d) Osteoclast precursors were differentiated in the presence of 50 ng ml−1M-CSF, 120 ng ml−1RANKL and the indicated concentrations of rhIGFBP5. Tartrate-resistant acid phosphatase (TRAcP) staining. Scale bar, 50 μm. (e) Count of TRAcP-positive multinucleated cells per well (mean±s.d.,n=4, **P<0.0002; *P<0.04, Student'st-test) in the cultures shown ind. (f) Osteoclasts obtained by M-CSF/RANKL treatment were detached and replated on bone sections in the presence of the indicated IGFBP5 concentrations to evaluate bone resorption by the pit index (mean±s.d.,n=3, *P<0.05, Student'st-test). (g) Sub- and overconfluent osteoblasts were treated with the indicated concentrations of IGFBP5 per 24 h. RT–PCR and relative quantification ofRanklandOpgexpression, normalized toGapdh, and their expression ratio (mean±s.d.,n=3, *P<0.05; **P<0.005;#P<0.01, Student'st-test). (h) Cartoon describing the amplification and inhibitory loops involving c-Src, IL-6 and IGFBP5 in immature osteoblasts, and the IGFBP5-dependent osteoblast-to-osteoclast cross-talk. (i) Cartoon describing the relationship between c-Src, Runx2 and IGFBP5 in mature osteoblasts, and the IGFBP5-dependent osteoblast-to-osteoclast cross-talk.Gapdh,glyceraldehyde-3-phosphate dehydrogenase. Figure 6: IGFBP5 effects on osteoblasts and osteoclasts. ( a ) Mouse calvarial osteoblasts were cultured at subconfluence and treated with the indicated concentrations of soluble IGFBP5 for 30 min. Western blot analysis of c-Src activating phosphorylation and total c-Src protein, normalized versus actin. ( b ) Mouse calvarial osteoblasts were cultured at overconfluence and treated with the indicated concentrations of soluble IGFBP5 for 30 min. Western blot analysis of c-Src activating phosphorylation and total c-Src protein, normalized versus actin. ( c ) ELISA assay for mIGFBP5 detection in the conditioned media from sub- and overconfluent osteoblasts treated with 5 ng ml −1 rhIL-6 or with 2 μM PP1 (mean±s.d., n =3. * P <0.05 and ** P <0.005, Student's t -test). ( d ) Osteoclast precursors were differentiated in the presence of 50 ng ml −1 M-CSF, 120 ng ml −1 RANKL and the indicated concentrations of rhIGFBP5. Tartrate-resistant acid phosphatase (TRAcP) staining. Scale bar, 50 μm. ( e ) Count of TRAcP-positive multinucleated cells per well (mean±s.d., n =4, ** P <0.0002; * P <0.04, Student's t -test) in the cultures shown in d . ( f ) Osteoclasts obtained by M-CSF/RANKL treatment were detached and replated on bone sections in the presence of the indicated IGFBP5 concentrations to evaluate bone resorption by the pit index (mean±s.d., n =3, * P <0.05, Student's t -test). ( g ) Sub- and overconfluent osteoblasts were treated with the indicated concentrations of IGFBP5 per 24 h. RT–PCR and relative quantification of Rankl and Opg expression, normalized to Gapdh , and their expression ratio (mean±s.d., n =3, * P <0.05; ** P <0.005; # P <0.01, Student's t -test). ( h ) Cartoon describing the amplification and inhibitory loops involving c-Src, IL-6 and IGFBP5 in immature osteoblasts, and the IGFBP5-dependent osteoblast-to-osteoclast cross-talk. ( i ) Cartoon describing the relationship between c-Src, Runx2 and IGFBP5 in mature osteoblasts, and the IGFBP5-dependent osteoblast-to-osteoclast cross-talk. Gapdh , glyceraldehyde-3-phosphate dehydrogenase . Full size image We then evaluated the IGFBP5 content in the conditioned media of sub- and overconfluent osteoblasts treated with IL-6 or PP1 for 24 h or 7 days, respectively. As shown in Fig. 6c , at subconfluence only the treatment with PP1 induced an increase of Igfbp5 , while at overconfluence this increase was found both in IL-6- and c-Src inhibitor-treated cultures compared with controls. Notably, basal Igfbp5 level at overconfluence was higher than at subconfluence, suggesting a spontaneous increase in this protein in mature osteoblasts. IGFBP5 was unable to affect adipogenesis as neither intensity of oil-red O staining ( Supplementary Fig. S2a ) nor PPARγ transcriptional expression ( Supplementary Fig. S2b ) were changed in IGFBP5-treated osteoblasts versus control cultures, both at sub- and overconfluence. As in mature osteoblasts IGFBP5 can no longer stimulate c-Src ( Fig. 6b ), we wondered if other cells of the bone microenvironment could be targeted by the protein. To test this hypothesis, we treated osteoclast precursors with IGFBP5 and assessed the rate of in vitro osteoclastogenesis. The results showed a robust increase in the number of osteoclasts generated in the presence of IGFBP5 ( Fig. 6d,e ). IGFBP5 also increased bone resorption ( Fig. 6f ) at an IGFBP5 concentration slightly higher than that necessary to stimulate osteoclast formation. Finally, IGFBP5 induced an increase in the receptor activator of nuclear factor-κB ligand (RANKL)/ Osteoprotegerin (OPG) ratio in subconfluent but not in overconfluent osteoblasts ( Fig. 6g ), suggesting the involvement of this pathway in the IGFBP5-dependent osteoblast–osteoclast cross-talk only at the early stage of osteoblast differentiation. Our findings showed a c-Src-mediated control of IL-6 transcription, both in vitro and in vivo . In fact, this tyrosine kinase is responsible, at least in part, for the activating phosphorylation of STAT3, which is a transcription factor for IL-6 and a component of the IL-6 signal. The cooperation between c-Src and STAT3 seems to have a biological relevance, as the modulation of both proteins determined similar effects on osteoblasts. Moreover, a feedback regulation of STAT3 on c-Src activation was established. Indeed, the canonical IL-6 signal, acting on STAT3 transcription factor, promotes the expression of genes involved in the activation of c-Src, among which we found the IGFBP5. In our proposed mechanism, c-Src could amplify the IL-6 signal through STAT3, inducing IL-6 gene expression ( Fig. 6h ). Secreted IL-6 could act in a paracrine or autocrine manner on osteoblasts, inducing its canonical pathway, again through STAT3 activation. Canonical STAT3 activation by IL-6 signal could induce the expression of IGFBP5, which is secreted in the bone microenvironment and could act on osteoblasts to induce c-Src-dependent non-canonical STAT3 activation ( Fig. 6h , amplification loop). In this instance, the cooperation between c-Src and STAT3 could delay osteoblast differentiation with a positive feedback between IL-6 and c-Src pathways. Consistent with our model, we demonstrated that IL-6 enhances the expression of Igfbp5 , which has been described to have important roles in bone physiology and pathology [19] , [20] , [21] , [22] . Interestingly, we found that IGFBP5 directly induced c-Src activation without affecting IGF-1 receptor phosphorylation. The mechanism by which IGFBP5 stimulates c-Src phosphorylation remains to be elucidated. Recent reports suggest that IGFBP5 can modulate cell metabolism by a putative IGFBP5 receptor [23] . However, there is no unequivocal evidence of its existence and nature, and some data in literature suggest that IGFBP5 has a negative role on osteoblast differentiation through its ability to bind IGF-1 (ref. 24 ). Our results seem to favour the possibility that, at least in our experimental conditions, IGFBP5 may exert its action on osteoblasts through a mechanism that does not require its binding to IGF-1. In the attempt to understand whether activated c-Src has also a role in the regulation of IGFBP5 activity, we have identified an additional regulatory loop. Unexpectedly, activated c-Src had an inhibitory role on IGFBP5 expression ( Fig. 6h , inhibitory loop). In fact, when we inhibited c-Src activity we observed a severalfold increase (instead of a decrease) of IGFBP5 mRNA and protein release in the conditioned media, which sharply contrasted with the effect of c-Src on IL-6-induced IGFBP5 expression. Reconciling these conflicting data has been possible when we observed that the Igfbp5 promoter is subjected to regulation by Runx2, which in turn is induced by c-Src inhibition. Indeed, overexpression of Runx2 and inhibition of c-Src have identical effects on Igfbp5 expression, both promoting IGFBP5 transcription. It is known that Yes-associated protein is a mediator of Src/Yes signalling to Runx2, suppressing its transcriptional activity [25] , thus representing a possible signal through which c-Src can downregulate Igfbp5 ( Fig. 6h ). When this signal is removed by c-Src inhibition, as occurs for instance in mature osteoblasts, Runx2 is activated and increases Igfbp5 expression ( Fig. 6i ). Indeed in overconfluent (mature) osteoblasts, Igfbp5 expression was high but it was no longer able to induce c-Src activation. In this study, we also identified an alternative target of IGFBP5 in the bone environment, the osteoclast. On the basis of our observations, we propose a model in which Igfbp5 produced by osteoblasts not only could be deposited in the newly forming bone matrix, but it could also enhance osteoclast formation and activity, thereby acting as an osteoblast–osteoclast coupling signal ( Fig. 6h,i ). In addition to these roles, in immature osteoblasts, Igfbp5 could contribute autocrinely to keep c-Src active and osteoblasts in a less differentiated status, and could further stimulate osteoclast activity via an increase of the RANKL/OPG ratio. The balance and the timing among these Igfbp5 effects could account for a fine-tuning regulation of osteoblast activity in the context of the IL-6 regulatory pathway. Our results showed that also in vivo there is a relationship between c-Src activity, IL-6 expression and IGFBP5. It appears that c-Src-mediated IL-6 regulation is detectable especially in the bone microenvironment. In fact, in physiological condition, in vivo c-Src inhibition caused a reduction of IL-6 expression in the bone tissue. Similarly, in inflammatory condition, c-Src inhibition was also able to downregulate IL-6 expression in the bone microenvironment. It is interesting to note that, in mice overexpressing human IL-6, in which the transgene is not modulated but is able to induce endogenous (mouse) IL-6 upregulation, c-Src inhibitor was again able to impair the expression of this latter in the tibia. Moreover, c-Src inhibition had a strong anabolic effect on the bone of IL-6 TG mice, in which osteoblasts are negatively affected by IL-6 overexpression [13] . It is also interesting that, in an animal model of bone metastases, c-Src inhibition strongly downregulated IL-6 derived from both the human metastatic cells and the mouse host tissues. A potential therapeutic impact could be predicted from these results, hypothesizing that a c-Src inhibitor could be used in cancer-induced bone diseases not only to impair osteoclast bone resorption and tumour cell proliferation [17] , [26] , [27] , but also to reduce IL-6 production and, therefore, its deleterious systemic effects on the body. Indeed, clinical trials are in progress for cancer using the c-Src inhibitor Saracatinib, which, in our opinion, associated with the IL-6 receptor-neutralizing antibody Tucilizumab, may open new avenues for combination treatment of patients. Cell cultures and treatments Primary mouse calvarial osteoblasts were obtained through the sequential collagenase/trypsin digestion method. Briefly, calvaria from 6- to 9-day-old CD1 mice were washed in sterile Hank's balanced salt solution and sequentially digested for 10, 20 and 40 min at 37 °C with gentle agitation in medium supplemented with 1 mg ml −1 type IV collagenase (Difco Laboratories) and 0.25% trypsin (Sigma-Aldrich). Cells released in the second and third digestions were collected by centrifugation (290 g ) and plated in Dulbecco's modified Eagle's medium (DMEM) supplemented with 10% fetal bovine serum, 4 mM L -glutamine, 5 IU ml −1 penicillin and 5 μg ml −1 streptomycin (Hyclone). Cultures were free of osteomacs contamination as assessed by histochemical staining for Tartrate-resistant acid phosphatase (TRAcP; Sigma-Aldrich; Supplementary Fig. S3 ). For oil-red O staining, cells were fixed with 10% formaldehyde for 60 min, with 60% isopropanol for 5 min, and then stained with oil-red O (Sigma-Aldrich) for 5 min at room temperature. Mouse bone marrow mononuclear cells were isolated from long bones of 6- to 9-day-old mice. The mononuclear cell fraction was isolated by centrifugation on Histopaque 1077 (Sigma-Aldrich) and cultured in 96-multiwell plates for 1 week in DMEM containing 10% fetal bovine serum, 50 U ml −1 penicillin, 50 μg ml −1 streptomycin, 2 mM L -glutamine, 50 ng ml −1 macrophage colony-stimulating factor (M-CSF) and 120 ng ml −1 soluble RANKL. Cultures were refreshed twice weekly. After 1 week, cells were fixed in 4% paraformaldehyde and stained for the osteoclast-specific marker, TRAcP. Osteoclasts were recognized by light microscopy as >3 nuclei containing TRAcP-positive giant cells. Nuclei were stained with Hoechst 3342. To evaluate bone resorption, differentiated osteoclasts were detached by standard trypsin procedure, cultured on bone slices for further 48 h, then removed by sonication before metachromatic staining of the slices with 1% toluidine blue. The formation of resorption pits was quantified by the pit index method. Briefly, the resorption pits were divided in three visual categories, according to their diameter: small, <10 μm; medium 10–30 μm; and large >30 μm. The numbers of pits per each category were scored by multiplying by a different factor according to their dimensions: for small pits, 0.3; for medium pits, 1; and for large pits, 3. The sum of the three scores gave the pit index [28] . Primary mouse osteoblasts were treated with PP1 (Calbiochem) for c-Src inhibition and with recombinant human IL-6 (R&D Systems). Primary mouse osteoblasts and osteoclasts were treated with soluble IGFBP5 (Abcam) for functional assays. All treatments were performed in cells starved for 24 h in serum-free medium. Transcriptome profiling For microarray analysis, sample labelling, hybridization and staining were carried out according to the Eukaryotic Target Preparation protocol in the AffymetrixR Technical Manual (701021 rev 1) for GeneChipR Expression Analysis (Affymetrix). Mouse MG-U74v2 arrays were scanned in an Affymetrix GeneChip scanner 3,000 at 570 nm. The final data set was obtained using the Affymetrix Microarray Suite 5.0 software. The significantly regulated genes were clustered using the web-based platform Gene Ontology Tree Machine, whose software uses statistical analysis indicating Gene Ontology terms with relatively enriched gene numbers and suggesting interesting biological areas. The microarray data have been deposited in the GEO database under the accession code GSE34570 . RT–PCR Total RNA was extracted from cultured cells using the standard Trizol procedure. For extraction from whole bones, total RNA was obtained by pestling the tibias in liquid nitrogen, followed by standard Trizol procedure. One μg of RNA was reverse transcribed using the Moloney murine leukaemia virus reverse transcriptase, and the equivalent of 0.1 μg was used for the PCRs. These were carried out in a final volume of 50 μl containing 200 μM of dNTPs, 1.5 mM MgCl 2 , 10 pM of each primer and 1 unit Taq DNA polymerase. Primer pairs and PCR conditions are shown in Supplementary Table S1 . For quantitative analysis, primers for the housekeeping gene Gapdh were used along with the primers for the gene being analysed. PCR-amplified products were analysed on 1% agarose gel containing ethidium bromide and subjected to densitometry by a Bio-Rad scanning densitometer (Bio-Rad, Hercules, CA), model GS800, equipped with Bio-Rad Quantity One image analysis software. RT–PCR reagents were from Invitrogen. Conditioned media and sera analysis The levels of mouse and human IL-6 were measured in culture supernatants and in sera of experimental animals by ELISA, using the mouse and the human IL-6 DuoSet ELISA Development Kit (R&D System), respectively, according to the manufacturer's instructions. Mouse IGFBP5 content was measured in the culture supernatants by ELISA, using the mouse IGFBP5 DuoSet ELISA Development Kit (R&D System). Osteocalcin, TRAP-5b and C-terminal fragment of Collagen I were evaluated in the sera of experimental animals using, the Mouse Osteocalcin EIA kit (Biomedical Technologies), the Mouse Trap Assay (Immunodiagnostic Systems) and the RatLaps EIA kit (Immunodiagnostic Systems) respectively, according to the manufacturer's instructions. Immunoprecipitation and western blotting Cells were lysed in radioimmunoprecipitation assay (RIPA) buffer, and protein content was measured by the Bradford method. For immunoprecipitation, 5 μg of specific antibodies or preimmune serum was incubated for 2 h at 4 °C with protein G-conjugated agarose beads. After five washes in RIPA buffer, 1 mg of protein of each sample was added and incubated overnight at 4 °C. Samples were then washed with RIPA buffer, resuspended in 2× reducing Laemmli sample buffer, and boiled before SDS–PAGE. For western blot, cells were lysed in Isotriton buffer containing protease inhibitors (1 mM sodium orthovanadate and 2.5 mM sodium fluoride (pH 7)). Supernatants were stored at −80 °C. A quantity of 20–40 μg of lysates were resolved by 10% SDS–PAGE and transferred to nitrocellulose membranes. Blots were probed with the primary antibody for the indicated proteins, overnight at 4 °C, washed and incubated with the appropriate horseradish peroxidase (HRP)-conjugated secondary antibody for 1 h at room temperature, subsequently detected with an enhanced chemoluminescence kit, according to the manufacturer's instructions. Anti-v-Src antibody was from Calbiochem (dilution 1:600). Antiphospho-Y416-Src (dilution 1:1,600) and antibodies against STAT proteins (dilution 1:1,100), IGF-1 receptor (dilution 1:1,000) and phospho-IGF-1 receptor (dilution 1:600) were from Cell Signaling Technology. Hybond-C extra nitrocellulose membranes and the enhanced chemoluminescence kit were from Amersham Bioscience. RNA interference knockdown of gene expression Four siGENOME SMART pool siRNA duplexes specific for mouse c-Src, STAT3 and IGFBP5 were purchased from Dharmacon. Osteoblasts were plated in 24-well plates or in 3.5-cm culture dishes. At ~50% confluence, cells were transfected with the annealed siRNA–c-Src and siRNA–STAT3 (siRNA final concentration 100 nM) using oligofectamine (Invitrogen). Cells were treated with siRNA for 48 h, then proteins were extracted and subjected to western blot to evaluate total protein expression. RNA was then extracted, reverse transcribed and subjected to PCR amplification for the genes of interest. Electroporation Pelleted cells were resuspended in fresh medium and counted, then sufficient cells for all transfections (1×10 6 cells per transfection) were transferred to a fresh tube and centrifuged at 200 g for 3 min. Cell aliquots were also retained from the cell suspension for use as non-transfected controls. After carefully removing the supernatant, the cell pellet was resuspended in 100 μl Mouse Primary Neurons Nucleofector Solution (Amaxa Biosystems) per transfection, then 100 μl was added to 2 μg of an empty vector (pmaxGFP; Amaxa Biosystems), WT and DN c-Src plasmids. The solution was added to Amaxa electrode cuvettes and electroporated in an Amaxa Nucleofector II using program Y-020. Immediately afterward, cells were diluted in 2.5 ml DMEM (supplemented with 20% FCS, 100 U ml −1 penicillin, 0.1 mg ml −1 streptomycin, 2 mM L -glutamine) at room temperature. Cells were then seeded onto dentine slices in 96-well plates (4×10 4 per well) and onto 9-mm glass coverslips in 48-well plates (1×10 5 per well). Non-transfected control cells were seeded at half of this density. Medium was replaced after 48 h with DMEM (+10% FCS, 100 U ml −1 penicillin, 0.1 mg ml −1 streptomycin, 2 mM L -glutamine). Immunostaining Primary mouse osteoblasts were isolated from neonatal calvarial bones, as described above, seeded in dishes containing glass coverslips, treated for 24 h with 2 μM PP1, then fixed in 4% formaldehyde. Cells were permeabilized by incubation with 0.2% Triton X-100 for 20 min, blocked with 1% BSA in PBS for 1 h, then incubated with 1:200 rabbit polyclonal STAT3 antibody (Cell Signaling Technology) or 1:100 rabbit polyclonal IGFBP5 antibody (Santa Cruz Biotechnology) in PBS/1% BSA for 1 h. Cells were washed three times in PBS, incubated with TRITC-anti-rabbit immunoglobulin-G (diluted 1:200) for 1 h, washed extensively again in PBS, then counterstained with 4,6-diamidino-2-phenylindole and analysed by fluorescence microscopy. Immunohistochemistry was performed to detect mouse or human IL-6 with species-specific anti-IL-6 antibodies (R&D System), mouse phospho-Y705-STAT3 (R&D System) and mouse IGFBP5 (Santa Cruz Biotechnology; all diluted 1:100), using the LSAB2 System-HRP kit (DAKO), according to the manufacturer's instructions. Animals All in vivo experiments were conducted in accordance with the principles and procedures outlined in the NIH (National Institute of Health) 'Guidelines and Care and Use of Experimental Animals' and in the Italian Legislative Decree 116/92, and were approved by our Ethical Board. C57 and Balb-c nu/nu immunocompromised mice were purchased from Charles River. IL-6 TG mice (cb6/f1 background) were previously generated using the NSE/hIL-6 construct, which carries the rat neurospecific enolase (NSE) promoter driving the expression of human IL-6 complementary DNA [29] . These mice show high circulating level of IL-6 since birth, significantly reduced growth rate, and normal food intake, haematic glucose and lifespan. Mice were housed in our animal facility with weekly veterinary check. C57 mice, IL-6 TG mice and their WT counterpart were subjected to treatment with 100 mg kg −1 c-Src inhibitor CGP76030 (Novartis) by oral gavage for 30 days. Groups of C57 mice were also treated with LPS (2.5 μg per mouse) or turpentine (100 μl per mouse) for 3 h to elicit inflammatory response. Balb-c nu/nu mice were injected intracardiacally with human breast cancer MDA-MB-231 cells and treated with 100 mg kg −1 CGP76030 by oral gavage 5 days per week for 38 days. At the end of the experiments, mice were euthanized by CO 2 inhalation and sera were collected to analyse IL-6 concentration by ELISA. Tibias were either fixed and embedded in paraffin for histological analyses or frozen and used for RNA extraction and IL-6 expression analysis by RT–PCR. Bone histology and histomorphometry Tibiae and femurs were fixed in 4% formaldehyde in 0.1 M phosphate buffer (pH 7.2), dehydrated in ethanol or acetone, and processed for paraffin embedding with previous decalcification or for glycol–methacrylate embedding without decalcification, respectively. Histomorphometric measurements were carried out on 2–5-μm-thick sections with an interactive image analysis system (IAS 2000; Delta Sistemi, Rome, Italy). Nomenclature, symbols and units of histomorphometric bone variables are those suggested by the Histomorphometry Nomenclature Committee of the American Society for Bone and Mineral Research. Statistics Data are expressed as the mean±s.d. of at least three independent experiments and five animals per group. Statistical analysis has been performed by the Student's t -test. P -values <0.05 have been considered statistically significant. Accession codes: The microarray data has been deposited in the GEO database under the accession code GSE34570 . How to cite this article: Peruzzi, B. et al . c-Src and IL-6 inhibit osteoblast differentiation and integrate IGFBP5 signalling. Nat. Commun. 3:630 doi: 10.1038/ncomms1651 (2012).